Mutually synchronized bottom-up multi-nanocontact spin–torque oscillators Spin–torque oscillators offer a unique combination of nanosize, ultrafast modulation rates and ultrawide band signal generation from 100 MHz to close to 100 GHz. However, their low output power and large phase noise still limit their applicability to fundamental studies of spin-transfer torque and magnetodynamic phenomena. A possible solution to both problems is the spin-wave-mediated mutual synchronization of multiple spin–torque oscillators through a shared excited ferromagnetic layer. To date, synchronization of high-frequency spin–torque oscillators has only been achieved for two nanocontacts. As fabrication using expensive top–down lithography processes is not readily available to many groups, attempts to synchronize a large number of nanocontacts have been all but abandoned. Here we present an alternative, simple and cost-effective bottom-up method to realize large ensembles of synchronized nanocontact spin–torque oscillators. We demonstrate mutual synchronization of three high-frequency nanocontact spin–torque oscillators and pairwise synchronization in devices with four and five nanocontacts. Spin–torque oscillators (STOs) [1] , [2] , [3] , [4] , [5] , [6] , [7] represent a novel class of nanoscopic microwave signal generators combining ultra-broadband operation [8] , [9] , [10] , ultrafast modulation [11] , [12] , [13] , [14] , [15] , [16] , an extremely small footprint, straightforward CMOS integration using commercial MRAM processes [17] , [18] , and potential for magnonic devices [19] , [20] , [21] , [22] , [23] , [24] . Their main drawbacks are their limited output power and high phase noise caused by tiny mode volumes and a strong frequency–power nonlinearity [25] , [26] , [27] , [28] . Although the solution lies in the mutual synchronization of several nanocontacts, this has only been achieved for two high-frequency nanocontact STOs [29] , [30] , [31] , [32] , [33] and four low-frequency vortex STOs [34] , all fabricated using either low-volume e-beam lithography or atomic force microscopy nano-indentation. The active area of a nanocontact STO is typically an extended giant magnetoresistance (GMR) trilayer on top of which one or several nanocontacts of the order of 100 nm diameter are fabricated. Each nanocontact can sustain several tens of mA current, which gets spin polarized and transfers angular momentum between the two magnetic layers via the so-called spin-transfer torque (STT) effect [35] , [36] , [37] . At sufficiently high current densities (~10 8 A cm −2 ), STT can sustain continuous precession of the local magnetization underneath the nanocontact and also inject high amplitudes of either localized or propagating spin waves (SWs) into the free layer [20] , [22] , [23] , [38] , [39] , [40] , [41] , [42] , [43] . Here we present a manufacturing technique that opens up the possibility to fabricate a variety of STT devices, specifically nanocontact STOs arrays, without expensive high-performance lithography equipment. By utilizing small polystyrene spheres, nanostructures with a wide range of sizes can be readily fabricated [44] . The structures are organized in an amorphous pattern, as the result of charged based short-range-ordering of nanoparticles with a wide tunable density. Using this technique, we have fabricated nanocontact STOs with single and multi-nanocontacts on a Co/Cu/Ni 81 Fe 19 GMR thin-film stack. A statistical analysis of the number of nanocontacts for 100 and 80 nm diameters is presented. The fabricated devices show mutual synchronization in STOs with up to three nanocontacts and pairwise synchronization in devices with four and five nanocontacts. Fabrication of nanocontact STOs The fabrication process begins with magnetron sputter deposition of a Pd (5 nm)/Cu (10 nm)/Co (5.5 nm)/Cu (4 nm)/Ni 81 Fe 19 (3 nm)/Cu (2 nm)/Pd (2 nm) GMR stack, using high-purity (>99.95 at%) stoichiometric targets in a confocal sputtering geometry, onto a thermally oxidized (1 μm SiO 2 ) 100 mm diameter Si wafer, in a chamber with a base pressure better than 1 × 10 −8 Torr. The thick Cu layer allows for a decreased resistance of the complete structure. It will in essence allow the current to flow perpendicularly to the plane through the spin valve. This effectively limits the current spread and enables spin–torque effects from nanocontact geometries [45] , [46] . Cobalt and permalloy (Ni 81 Fe 19 ) are the fixed and free layer, respectively. To induce a magnetic easy axis, a magnetic field of 300 Oe was applied in the film plane during deposition. Photoresist, I-line (365 nm) stepper photolithography (Ultratech XLS 7500/2145) and an Applied Materials Precision 5000 Mark II argon plasma etching system was used to pattern the GMR stack into 8 × 16 μm 2 mesas. After removing the photoresist in a two-step process of a short oxygen plasma and Microposit 1165 resist remover, the structures were covered with 30 nm of SiO 2 and deposited in a plasma-enhanced chemical vapour deposition system. A combination of hole-mask colloidal lithography [44] and optical lithography was used to fabricate the nanoholes through the SiO 2 . The wafer was spin-coated with poly-(methyl methacrylate) (PMMA), which acts as a mask when the nanoholes are etched out in the SiO 2 . A short O 2 plasma ashing process improved the hydrophilicity of the PMMA. After this, a polyelectrolyte solution was distributed onto the surface using a pipette, forming positive surface charges that attract the negatively charged polystyrene spheres later poured as a suspension on top of the PMMA and the polyelectrolyte adhesion layer. The negative charge promotes separation in between spheres and adhesion to the surface. The spheres are suspended in a deionized (DI) water-based solvent that is rinsed with (DI) water after 2 min on the surface. Blow drying by nitrogen was employed to assist DI water evaporation and to avoid rearrangement of the spheres on the surface. Spheres, 20–120 nm in diameter, can be utilized in the method ( Fig. 1a ). A thin, 10-nm chromium film was deposited by e-beam evaporation on top of the spheres to function as a hard mask for subsequent etching of the PMMA ( Fig. 1b ). By first attaching an adhesion tape (SWT-10 tape, Nitto Scandinavia AB) ( Fig. 1c ) that adheres to the top of the chromium-covered spheres and then removing the tape, a chromium film with a multitude of nanoholes on top of the PMMA ( Fig. 1d ) was realized. To achieve a limited number of nanoholes (and subsequent nanocontacts) per device, a second photolithography step was introduced, called a ‘limiter mask’ ( Fig. 1e ). The wafer was put in a directional oxygen plasma that etches the PMMA anisotropically, forming vertical channels down to the SiO 2 . Due to to the thickness difference between PMMA (120 nm) and photoresist (1,500 nm), the photoresist remained during this step ( Fig. 1f ). The SiO 2 was then etched in an RIE Oxford system with Ar (10 sccm) and CHF 2 (20 sccm) plasma with a total pressure of 30 mTorr and a power of 200 W ( Fig. 1g ). This recipe selectively etches the SiO 2 without affecting the material stack. Next, PMMA, chromium and resist were removed by a resist-remover step (Microposit 1165) leaving nanoholes in the SiO 2 film ( Fig. 1h ). A resist and etch step is added to open up larger areas in the SiO 2 layer on each side of the area of nanoholes. Contact to the nanoholes and the two ground contacts are achieved using a 1-μm thick Ag ground-signal-ground waveguide, deposited using electron beam evaporation and patterned using optical lithography and lift off. 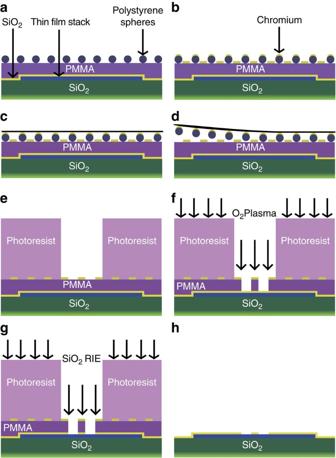Figure 1: Nanohole fabrication process. (a) Covering the mesa with SiO2, PMMA and placing the polystyrene spheres on the surface. (b) Chromium mask evaporation (c) placing adhesion tape, (d) removing the tape and the spheres, (e) limiter mask, photolithography step, (f) directional oxygen plasma, (g) SiO2etching and (h) resist strip. Figure 1: Nanohole fabrication process. ( a ) Covering the mesa with SiO 2 , PMMA and placing the polystyrene spheres on the surface. ( b ) Chromium mask evaporation ( c ) placing adhesion tape, ( d ) removing the tape and the spheres, ( e ) limiter mask, photolithography step, ( f ) directional oxygen plasma, ( g ) SiO 2 etching and ( h ) resist strip. Full size image Being able to control the number, density and spacing of the nanocontacts is crucial for synchronized STO arrays, where the region of strong SW interaction typically extends a limited distance from the perimeter of the nanocontact [32] . 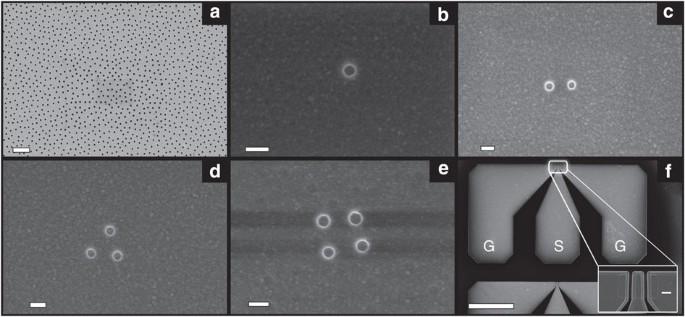Figure 2: Schematic sample layout. Scanning electron microscopy images. (a) Top view of chromium and PMMA mask (scale bar, 1 μm). (b–e) Single, double, triple and quadruple 100 nm nanoholes in SiO2made through a (b–d) 500 nm opening (scale bar, 200 nm) and a (e) 600-nm opening on top of the GMR stack (scale bar, 200 nm). (f) Top contact waveguide for microwave measurements: signal (S) and two ground (G) pads are shown in the picture (scale bar, 100 μm); inset, magnified images of pad connection to the mesa (scale bar, 4 μm). Figure 2b–e show examples of how this process leads to one to four equally spaced nanoholes in SiO 2 . The final device, with a waveguide connecting to the nanocontact region and the ground contacts, is shown in Fig. 2f . Figure 2: Schematic sample layout. Scanning electron microscopy images. ( a ) Top view of chromium and PMMA mask (scale bar, 1 μm). ( b – e ) Single, double, triple and quadruple 100 nm nanoholes in SiO 2 made through a ( b – d ) 500 nm opening (scale bar, 200 nm) and a ( e ) 600-nm opening on top of the GMR stack (scale bar, 200 nm). ( f ) Top contact waveguide for microwave measurements: signal (S) and two ground (G) pads are shown in the picture (scale bar, 100 μm); inset, magnified images of pad connection to the mesa (scale bar, 4 μm). Full size image Nanocontact statistics The degree of achievable multi-nanocontact control is presented in Fig. 3 , which shows the distribution of nanocontacts for different diameters of the limiting mask and for two different concentrations of the suspension. Eighteen nanocontact STO devices were analysed for each fabrication condition. At the highest concentration of spheres, the smallest limiter (0.45 μm) results predominantly in double nanocontacts (55%) with some fraction of both single (28%) and triple (17%) nanocontacts. As the size of the limiting mask is increased, the number of nanocontacts per device increases, with the largest opening (0.8 μm) yielding devices having over ten nanocontacts. As can be seen in Fig. 3b,c , a lower concentration of spheres shifts the distributions to fewer nanocontacts per device. For example, in Fig. 3c , the smallest limiter (0.5 μm) results predominantly in single nanocontacts (55%) and one fifth of all devices are without nanocontacts altogether. 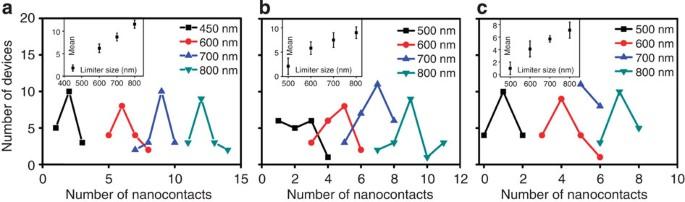Figure 3: Distributions of number of nanocontacts as a function of limiting mask diameter. (a) High concentration (0.04% w/v) of 80 nm spheres, (b) low concentration (0.02% w/v) of 80 nm spheres and (c) low concentration (0.02% w/v) of 100 nm spheres. Legend denotes the diameter of the limiting mask. Insets show the mean number of nanocontacts versus limiting mask diameter. Error bars indicate the full range of the data set. Figure 3: Distributions of number of nanocontacts as a function of limiting mask diameter. ( a ) High concentration (0.04% w/v) of 80 nm spheres, ( b ) low concentration (0.02% w/v) of 80 nm spheres and ( c ) low concentration (0.02% w/v) of 100 nm spheres. Legend denotes the diameter of the limiting mask. Insets show the mean number of nanocontacts versus limiting mask diameter. Error bars indicate the full range of the data set. Full size image Microwave characterization All devices with one or more nanocontacts showed microwave signal generation in a 1 Tesla magnetic field applied at 70° from the film plane when driven with sufficiently large currents ( I dc ). 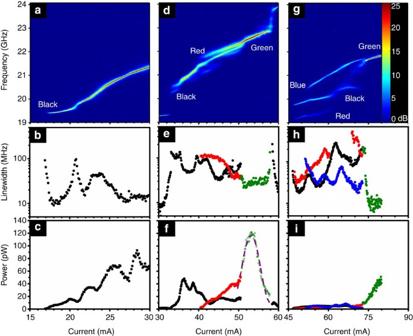Figure 4: STO signal properties as a function of current. Devices with single (a–c), double (d–e) and triple (g–i) nanocontacts. Green data points in the linewidth and power plots indicated a synchronized state. The dashed purple line infis a calculation of the expected power in the synchronized state based on equation (1). The colour labels ina,dandgrefer to the colours used in the linewidth and power plots. Figure 4 shows power spectral density colour maps versus I dc for three representative nanocontact STOs with (a) single, (d) double and (g) triple nanocontacts with nominal diameter of 100 nm. 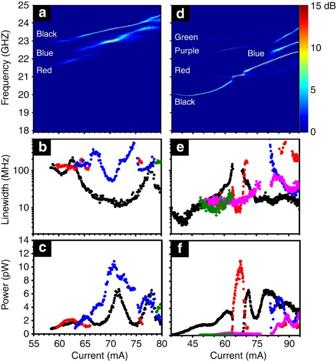Figure 5: STO signal properties as a function of current. Devices with (a–c) four- and (d–f) five-nanocontacts showing pairwise synchronization. The labels inaanddrefer to the colours used in the linewidth and power plots. Figure 5 shows the corresponding power spectral density maps and extracted microwave signal properties for a four- and a five-nanocontact STO. The generated signal from each nanocontact in Figs 4a,d,g and 5a,d is marked with a colour tag that identifies the corresponding linewidth in Figs 4b,e,h and 5b,e , and power in Figs 4c,f,i and 5c,f . It is noteworthy that the critical threshold current for microwave generation ( I th ) scales linearly with the number of nanocontacts, consistent with a constant critical current density independent of the number of nanocontacts. The single nanocontact STO starts oscillating at ~17 mA ( Fig. 4a ), the two-nanocontact STO starts at ~33 mA ( Fig. 4d ), the three-nanocontact STO starts at ~48 mA ( Fig. 4h ) and the first four-nanocontact STO starts at ~58 mA ( Fig. 5a ), consistent with I th =15–17 mA (per nanocontact) in all four devices (a current density of ~2 × 10 8 A cm −2 ). In a second four-nanocontact STO (not shown) and the five-nanocontact STO, the individual nanocontacts show a larger spread in threshold currents, which may reflect some variation in nanocontact size. Figure 4: STO signal properties as a function of current. Devices with single ( a – c ), double ( d – e ) and triple ( g – i ) nanocontacts. Green data points in the linewidth and power plots indicated a synchronized state. The dashed purple line in f is a calculation of the expected power in the synchronized state based on equation (1). The colour labels in a , d and g refer to the colours used in the linewidth and power plots. Full size image Figure 5: STO signal properties as a function of current. Devices with ( a – c ) four- and ( d – f ) five-nanocontacts showing pairwise synchronization. The labels in a and d refer to the colours used in the linewidth and power plots. Full size image The frequency generally blue shifts with increasing I dc , with the same current density dependence in all devices, which is consistent with the generation of a propagating SW mode with similar characteristics, regardless of the nanocontact number [22] , [24] , [32] . In the single nanocontact STO, a maximum total power of 95 pW is reached at ~28 mA, where the device also exhibits its narrowest linewidth of about 10 MHz ( Fig. 4c ). In the two- and three-nanocontact STOs, complete mutual synchronization can be observed at essentially the same current density (3.2 × 10 8 A cm −2 ) accompanied by a strong increase in power and a reduction in linewidth. The narrowest (5 MHz) linewidth of any device in this study is indeed observed for the fully synchronized three-nanocontact STO in Fig. 4h . Although none of the four- and five-nanocontact STOs showed complete synchronization, pairwise synchronization was readily observed, with a similar partial improvement in power and linewidth. Figure 5a shows a four-nanocontact STOs made with 0.6 μm limiter masks. The signals interact strongly with each other and get locked and unlocked a number of times, for example, between 65 and 78 mA in Fig. 5a for the signals at higher frequency (marked as black) and between 67 and 75 mA for the signal pair with lower frequency (blue and red). In many of these regions, the total power exhibits a cosine-like current dependence similar to the synchronized double nanocontact device. Gyrotropic vortex motion The nanocontact STOs presented in this study can also sustain gyrotropic vortex motion [47] , [48] , generating frequencies primarily below 1 GHz and showing operation in zero applied magnetic field [49] . Whereas we have not investigated the gyrotropic motion in detail, we here present an example of such operation. As can be seen in Fig. 6a , the device shows multiple harmonics and weak current tunability of 5.6 MHz mA −1 between 5 and 15 mA, which changes to 37 MHz mA −1 between 15 and 30 mA. A lowest linewidth of ~6 MHz was recorded at a drive current of 6 mA ( Fig. 6b ). In the region of stronger tunability, the linewidth increases to ~30 MHz ( Fig. 6b ). As known for these types of oscillation, the integrated power is much larger than for the propagating mode [34] . Although the power of the propagating SW mode generated by a single nanocontact barely reaches 100 pW, the vortex motion results in almost a 25-nW signal in the same device ( Fig. 6c ). 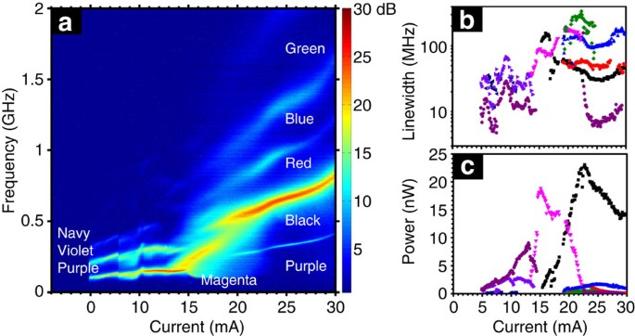Figure 6: STO vortex dynamic signal properties as a function of current. Single nanocontact device current scan in zero external field. (a) Current scan with multi-harmonics and mode changes. (b) Corresponding linewidth (c) integrated power. The labels inarefer to the colours used in the Linewidth and power plots. Figure 6: STO vortex dynamic signal properties as a function of current. Single nanocontact device current scan in zero external field. ( a ) Current scan with multi-harmonics and mode changes. ( b ) Corresponding linewidth ( c ) integrated power. The labels in a refer to the colours used in the Linewidth and power plots. Full size image It is interesting to note that the current-dependent power in the synchronized states exhibits a maximum in the centre of the synchronized region and a cosine-like fall-off when approaching either limit of this region ( Fig. 4f ). From the measured total microwave power of each signal just before synchronization ( p 1 =17 pW and p 2 =45 pW), we can calculate the power expected in the mutually synchronized state using the formula: where ϕ is the relative phase shift between the two nanocontacts. The maximum calculated power ( ϕ =0) of 117 pW is essentially identical with the measured maximum of 120 pW at 53.5 mA. We also find that a linear current dependence of ϕ approximates the experimental data quite well on both sides of this maximum (dashed purple line in Fig. 4f ). Whereas equation (1) can in principle be expanded to multi-nanocontacts, its application requires knowledge about all relative phase shifts ϕ . If we, for simplicity, assume that all three nanocontacts synchronize in phase at some point (maximum possible power), we can still apply the procedure above and use the three individual microwave power levels just before synchronization ( p 1 =7.0 pW, p 2 =1.7 pW and p 3 =1.4 pW) to predict the maximum microwave power in the synchronized state (26 pW). However, our measured maximum value, 47 pW ( Fig. 4i ), is almost twice as large as the prediction. The difference may very well be even greater, as the three-nanocontact STO cannot sustain high-enough currents to confirm that we have reached a true maximum. We ascribe this discrepancy to destructive interactions between the individual nanocontacts before synchronization, which reduces their individual power levels on approach to synchronization. Such a gradual deterioration can indeed be observed in Fig. 4g , where the overall coherence is low just before the three nanocontacts snap into their mutually synchronized state. In the parallel electrical connection of the multi-nanocontacts in our devices, the power delivered to the 50-Ω measurement load by N individually oscillating nanocontacts is expected to drop as N −2 due to the other nanocontacts acting as shunts [50] (see also Supplementary Note 1 ). When comparing the typical non-synchronized power of one through five-nanocontact STOs in Figs 4 and 5 , we clearly observe a dramatic reduction in power with the number of nanocontacts. For the same shunting reason, the maximum synchronized power delivered to the instrument should no longer scale with N 2 but be independent of N , that is, we expect the same extracted power from a single nanocontact STO as from any fully synchronized multi-nanocontact STO. This is clearly observed in Fig. 4 , where the synchronized state of two- and three-nanocontact STOs is of the same order as that of a single nanocontact STO. For parallel synchronization of multi-nanocontact STOs to provide a benefit not only in terms of linewidth but also in delivered microwave power, it is hence crucial to match the load or amplifier stage to the lower impedance of multi-nanocontact STOs compared with single nanocontact STOs [46] . The lack of complete synchronization in the four- and five-nanocontact STOs is likely due to a combination of two independent effects. First, whereas mutual synchronization in both two- and three-nanocontact STOs starts at a current density of ~3.18 × 10 8 A cm −2 , it is virtually impossible to reach the same value in devices with more than three nanocontacts before the nanocontact STO is destroyed. Although the maximum current density that these nanocontact STOs can sustain for enough measurement time before catastrophic failure is ~4.45 × 10 8 , 3.81 × 10 8 and 3.31 × 10 8 A cm −2 for one-, two- and three-nanocontact STOs, respectively; the four-nanocontact STO already breaks down at a current density of ~2.54 × 10 8 A cm −2 , that is, well before the current density required for complete synchronization is reached. The observed decreasing trend of the maximum sustainable current density indicates that it is, to an increasing degree, the total current and not the current density that limits the operating region, indicating that total heating in the larger combined nanocontact region and not in each nanocontact has an increasingly important role as the number of nanocontacts grows. Second, it is quite possible that the random nanocontact arrangement favours pairwise synchronization instead of complete synchronization. For randomly placed multi-nanocontacts, the SW pattern mediating the interaction between individual nanocontacts is expected to be much more complex and unpredictable than for only two nanocontacts. The system may hence very well find local optima (pairwise synchronization), while being unable to enter into a global optimum of complete mutual synchronization, similar to the so-called clustered synchronization in multi-oscillator systems [51] , [52] . In conclusion, we have presented a versatile and high-volume approach to the fabrication of single- and multi-nanocontact STOs without expensive and time-consuming e-beam or atomic force microscopy indentation-based lithography. By using different suspensions of polystyrene spheres, we fabricated a wide range of nanocontact STOs and demonstrated mutual synchronization in two- and three-nanocontact STOs, and pairwise synchronization in four- and five-nanocontact STOs. We believe that such a massively parallel and largely affordable bottom-up approach will drastically improve the accessibility of nanocontact-based spin–torque devices, which in turn will speed up the necessary improvement in material reliability to reach high-enough current densities for complete synchronization in large arrays of nanocontact STOs [13] , [14] , [15] , [16] . Measurement setup and condition In all the presented measurements, the positive current is defined as electrons entering the nanocontact from above and traversing the GMR stack from the NiFe free layer to the Co fixed layer. An external magnetic field with magnitude of 1 T was applied at 70° with respect to the sample plane and along the long direction of the GMR mesa. Direct current was provided to the samples with a Keithley 6221 current source and the sample voltage was monitored with a Keithley 2182 nanovoltmeter. A Bias-T was used to apply direct current only to the device, while allowing the generated microwave signal to pass through to a low noise amplifier (gain of 40 dB; bandwidth of 0.1–26.5 GHz) for final detection using a Rohde & Schwarz FSU 67 spectrum analyser (see Supplementary Fig. S1 ). Experimental data analysis The experimental data at each operating point (current, field) are recorded as a power spectral density acquired by a spectrum analyser. Each spectrum is fitted using one or more Lorentzian functions, and each Lorentzian is associated with one of the nanocontacts in the non-synchronized case. The Lorentzian fit is described by a peak frequency, a peak linewidth and a total integrated power under the Lorentzian peak. In Fig. 4 both for the double and triple nanocontact devices, we have used the last extracted power when all the two or three peaks were observed at their own individual frequencies. How to cite this article: Sani, S. et al. Mutually synchronized bottom-up multi-nanocontact spin–torque oscillators. Nat. Commun. 4:2731 doi: 10.1038/ncomms3731 (2013).